High-coherence picosecond electron bunches from cold atoms Ultrafast electron diffraction enables the study of molecular structural dynamics with atomic resolution at subpicosecond timescales, with applications in solid-state physics and rational drug design. Progress with ultrafast electron diffraction has been constrained by the limited transverse coherence of high-current electron sources. Photoionization of laser-cooled atoms can produce electrons of intrinsically high coherence, but has been too slow for ultrafast electron diffraction. Ionization with femtosecond lasers should in principle reduce the electron pulse duration, but the high bandwidth inherent to short laser pulses is expected to destroy the transverse coherence. Here we demonstrate that a two-colour process with femtosecond excitation followed by nanosecond photoionization can produce picosecond electron bunches with high transverse coherence. Ultimately, the unique combination of ultrafast ionization, high coherence and three-dimensional bunch shaping capabilities of cold atom electron sources have the potential for realising the brightness and coherence requirements for single-shot electron diffraction from crystalline biological samples. Ultrafast electron diffraction (UED) enables the study of molecular structural dynamics with atomic spatial resolution at picosecond timescales [1] , [2] , [3] . Determination of the structure and function of molecules is critical to understand all but the most simple chemical reaction pathways, to understand biochemical dynamics such as protein folding and regulation or to understand the formation of cracks in novel materials [4] , [5] . Progress with UED is constrained by the brightness and coherence of available electron sources. High-brightness electron beams for UED are typically generated from photocathodes [5] , [6] , [7] , [8] . The comparatively small inherent transverse coherence length of such sources is effectively increased by beam expansion with propagation and a beam aperture, according to the van Cittert-Zernike theorem [9] . The beam current is sacrificed for a reduced angular spread, effectively trading brightness for coherence length. Large increases in brightness are required for single-shot imaging of weakly scattering materials [5] . Cold atom electron sources (CAESs), which produce electrons by photoionization of laser-cooled atoms, promise to deliver the brightness and coherence required [10] for UED. Cold atom sources have generated electron bunches with high coherence, up to 10 nm at the source [11] . The bunch charge can be a few picocoulombs, sufficient for single-shot imaging of nanocrystals of biomolecules [12] , [13] , but the nanosecond duration of the electron bunches has been too long for observation of useful dynamics. With a cold atom source, electrons are typically produced by photionization of cold atoms in a two-step process, with microsecond laser excitation to an intermediate atomic state and nanosecond ionization of the excited atoms [11] , [13] . Time-dependent extraction fields can be used to reduce the electron bunch length [14] , but picosecond switching times are not feasible. A short ionization laser pulse could in principle produce a short electron bunch, but as the pulse duration Δ t is reduced, the spectral width of the pulse Δ ω must increase. At first glance, one might expect the energy uncertainty of the ionization pulse to be transferred to the electron momentum spread, thus reducing the transverse coherence. Here we show that, counter-intuitively, it is possible to generate electron pulses that are both short and coherent, using a femtosecond laser in a two-colour sub-threshold photoionization scheme. The femtosecond laser pulse is used to excite the cold atoms, and a comparatively long (nanosecond) laser pulse is used to photoionize the excited atoms. The laser pulses are temporally overlapped to produce short electron pulses with a static extraction field. With femtosecond excitation, the initial electron pulse duration is limited by the spatial extent of the overlap of the cold atoms and the two laser pulses, corresponding to around 150 ps for our apparatus (see Methods). Although that pulse duration is already short enough to observe the structural dynamics of a myoglobin mutant protein [4] , it may be possible to reduce the bunch length by up to three orders of magnitude using recently demonstrated radio frequency compression techniques [7] , [15] , [16] . Generation of cold electron bunches Experimentally, we extract cold electron bunches from laser-cooled rubidium atoms (see Fig. 1 ) with a repetition rate of 10 Hz. The excitation laser is either a switched on-resonant laser (50 ms duration) or a pulse from an 800-nm 35-fs laser system. In both cases, the excited atoms are ionized with a 5-ns 480-nm laser pulse and the bunches are extracted electrostatically. The experimental sequence involves loading a magneto-optic trap (90 ms) before extinguishing the cooling lasers and magnetic fields required for trapping and slowing the atoms (5 ms), then performing the ionization. A static electric field accelerates the electrons to an energy of 1 keV. For femtosecond excitation, the femtosecond pulse arrives at the atom cloud during the 5-ns ionization pulse. The relative delay is adjusted to optimize the detected electron intensity. The duration of the excitation laser pulse was determined to be 35 fs at the laser and 110±1 fs at the position of the atoms using frequency resolved optical gating [17] . 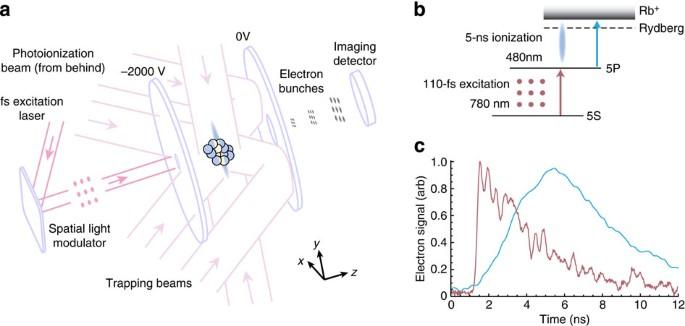Figure 1: CAES. (a) Schematic representation of the experimental setup11. A shaped 110-fs laser pulse is used to excite a pepper-pot distribution of atoms in thex–yplane, which are subsequently photoionized by a 5-ns laser pulse focused using a cylindrical lens to select a source plane. The electrons are accelerated for 2.5 cm by a 40 kV m−1electric field, expand under free propagation for 21.5 cm and are imaged using a phosphor-coupled microchannel plate (MCP) detector. (b) Simplified energy-level structure of rubidium. (c) MCP voltage (front ground plane) as electron pulses are detected, for femtosecond excitation (red)and for microsecond excitation (blue). Figure 1c shows the electron signal for pulses produced from both femtosecond and microsecond excitation. The signal shows a fast rise indicative of the short electron pulse duration and the bandwidth of the detector. The long decay is the same for all measurements, characterized by the detector response function. The 10/90 rise time with femtosecond excitation is 260 ps, much less than the 3.7 ns for the nanosecond pulse and clearly not limited by the 5P 3/2 lifetime of 25.8 ns. Based on the 100 μm full-width at half-maximum (FWHM) overlap of the cold atoms and laser pulses and the 40 kV m −1 field, we expect a minimum pulse length of 150 ps (see Methods). Figure 1: CAES. ( a ) Schematic representation of the experimental setup [11] . A shaped 110-fs laser pulse is used to excite a pepper-pot distribution of atoms in the x–y plane, which are subsequently photoionized by a 5-ns laser pulse focused using a cylindrical lens to select a source plane. The electrons are accelerated for 2.5 cm by a 40 kV m −1 electric field, expand under free propagation for 21.5 cm and are imaged using a phosphor-coupled microchannel plate (MCP) detector. ( b ) Simplified energy-level structure of rubidium. ( c ) MCP voltage (front ground plane) as electron pulses are detected, for femtosecond excitation (red) and for microsecond excitation (blue) . Full size image Two-colour and multi-photon ionization The laser pulses can drive photoionization through two processes: multi-photon and two-colour. Multi-photon ionization with an intense 800 nm, 110 fs laser pulse alone (that is, without the nanosecond laser) will produce ‘hot’ photoelectrons with a range of energies, due to the large bandwidth (measured as 20.4 nm) and many resonantly enhanced multi-photon ionization (REMPI) channels in the 770–830 nm band [18] . On the other hand, it has been shown [19] that the 5S 1/2 →5P 3/2 transition is coherently coupled when driven with a femtosecond laser pulse centred on λ =800 nm. With the addition of a 480 nm laser pulse, the 5P 3/2 state is coupled to the ionization continuum, or to high-lying Rydberg states, in a two-colour process. 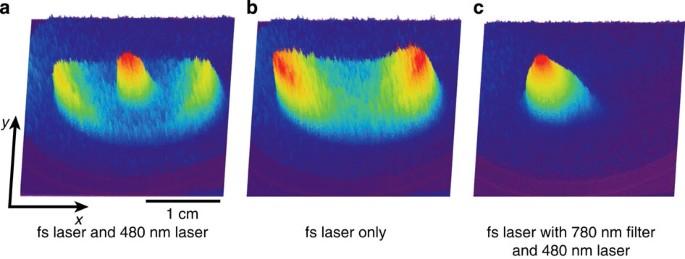Figure 2: Multi-photon and two-colour photoionization. False-colour three-dimensional representations of the photoelectron density signals as detected on the MCP. Ionization laser wavelengthλ=478.07 nm and pulse energy 800 μJ. Excitation laser 110 fs 20 μJ focused to 1 mm spot size. Each image is a 10-shot average of the electron signal. (a) Both the multi-photon and two-colour photoelectrons are visible. (b) Only the multi-photon photoelectrons are visible. (c) With excitation by aλ=780±1.5 nm filtered femtosecond pulse, only the two-colour photoelectrons are visible. Figure 2a shows the spatial distribution of detected ‘hot’ and ‘cold’ photoelectrons produced by multi-photon and two-colour ionization processes. Multi-photon ionization results in dipolar emission of hot photoelectrons in the plane of laser polarization, which are seen at large distances (momenta) from the beam axis, and cold photoelectrons produced from two-colour photoionization, seen as a central peak in the electron density. In Fig. 2b , the nanosecond ionization pulse is absent, and only hot REMPI photoelectrons are seen. If a λ =780±1.5 nm filter is placed in the femtosecond laser beam, multi-photon ionization is reduced, and the proportion of electrons produced by two-colour photoionization is enhanced; see Fig. 2c . Following these measurements to characterize the two photoionization processes, the 780-nm filter was removed from the femtosecond laser path, the 480 nm ionization pulse energy was set high enough to ensure that 5P 3/2 to continuum transition was saturated (3–20 mJ) and the pulse energy of the femtosecond laser was reduced until the REMPI signal was not significant (2 μJ). Figure 2: Multi-photon and two-colour photoionization. False-colour three-dimensional representations of the photoelectron density signals as detected on the MCP. Ionization laser wavelength λ =478.07 nm and pulse energy 800 μJ. Excitation laser 110 fs 20 μJ focused to 1 mm spot size. Each image is a 10-shot average of the electron signal. ( a ) Both the multi-photon and two-colour photoelectrons are visible. ( b ) Only the multi-photon photoelectrons are visible. ( c ) With excitation by a λ =780±1.5 nm filtered femtosecond pulse, only the two-colour photoelectrons are visible. Full size image Demonstration of low emittance and high transverse coherence The above measurements have demonstrated that a high bandwidth laser pulse can be used to reduce the electron pulse duration. Counter-intuitively, the two-colour femtosecond ionization process maintains high transverse coherence and high beam quality, despite the high bandwidth of the ultrafast laser pulse. The beam quality can be quantified by the transverse brightness and coherence length. Both are critical to UED and can be determined from the emittance, a measure of the phase-space volume occupied by the electron bunch (see Methods). To measure the emittance, we used the pepper-pot technique; that is, by measuring the transverse velocity spread as a function of position across the bunch. Typically, the pepper-pot distribution is created using a physical mask in the electron beam. The shaping capability of a CAES [11] removes the need for a mask, so that source diagnostic measurements can be performed without beamline alterations. The collection of electron ‘beamlets’ that forms a pepper-pot distribution was created with a shaped excitation laser pulse, and an ionization pulse focused in one dimension to form a ribbon. The spatial distribution of the propagated electron beamlets was measured at the detector, and emittance values were extracted following the method of Zhang [20] . Knowledge of the electron distribution in two planes (the photoionization and detection planes) provides the angular divergence of each beamlet, and, together with the propagation geometry, allows for direct calculation of the emittance ε r . The emittance values from a sequence of 50 single-shot measurements, such as that in Fig. 3 , were acquired and averaged, and uncertainties were calculated from the combination of systematic errors and the statistical deviation of the 50 values. 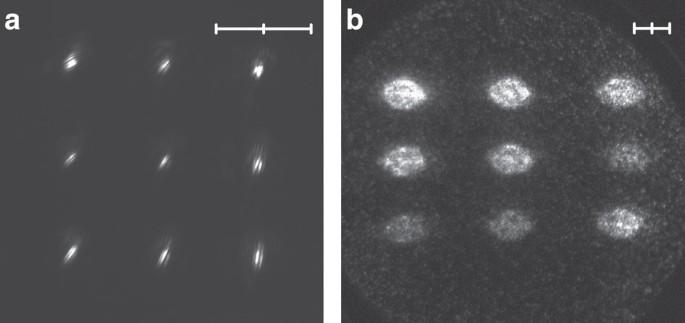Figure 3: Pepper-pot emittance measurement using optical pattern formation. Typical pepper-pot images used to extract the emittance of femtosecond-excited CAES electron bunches. (a) A CCD image of the laser pulse used to excite the atom cloud. (b) Detected electron signal for an ionization wavelength ofλ=478.00 nm. Scale bars, 2 mm. Figure 3: Pepper-pot emittance measurement using optical pattern formation. Typical pepper-pot images used to extract the emittance of femtosecond-excited CAES electron bunches. ( a ) A CCD image of the laser pulse used to excite the atom cloud. ( b ) Detected electron signal for an ionization wavelength of λ =478.00 nm. Scale bars, 2 mm. Full size image The emittance has two main contributions: thermal processes during ionization and extraction, and any excess energy imparted from the ionization laser. 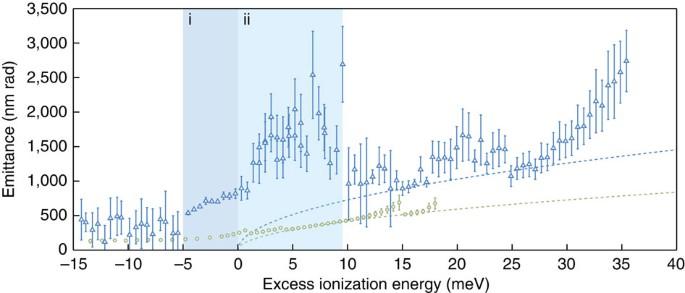Figure 4: Measured CAES emittance. The radial emittance is plotted as a function of excess ionization energy (given by equation (1)), beginning with the onset of electron production at the saddle-point energyEsp=−15.2meV, for picosecond (blue) and nanosecond (green) bunches. Each point represents the mean of 50 single-shot measurements with one s.d. error bars combined from the statistical deviation of the 50 shots and systematic uncertainties. Below −5 meV, the ionization efficiency is poor, reflected in the large error bars. In region i, the atoms are excited to a Rydberg state and field ionized. In region ii, just above the field-free threshold, we see rapid growth in emittance for femtosecond excitation. The dashed lines are theoretical emittance plots calculated from equation (6) (see Methods). Figure 4 shows the measured emittance values as a function of excess ionization energy. The excess energy Δ E ( λ ) is the difference between the field-free ionization energy hc / λ 0 and the laser energy, hc / λ : Figure 4: Measured CAES emittance. The radial emittance is plotted as a function of excess ionization energy (given by equation (1)), beginning with the onset of electron production at the saddle-point energy E sp =−15.2meV, for picosecond (blue) and nanosecond (green) bunches. Each point represents the mean of 50 single-shot measurements with one s.d. error bars combined from the statistical deviation of the 50 shots and systematic uncertainties. Below −5 meV, the ionization efficiency is poor, reflected in the large error bars. In region i, the atoms are excited to a Rydberg state and field ionized. In region ii, just above the field-free threshold, we see rapid growth in emittance for femtosecond excitation. The dashed lines are theoretical emittance plots calculated from equation (6) (see Methods). Full size image The energy threshold for ionization is lowered by the external electric field. The potential experienced by the electron is given by (in atomic units) −1/ r−Fz , where r the electron-ion separation, F is the external field strength and z is the distance along the field. That is, the ionization potential is lowered only in the z direction. Electrons are only produced when the energy is greater than the saddle-point energy, namely for F =40 kV m −1 . Between E sp <Δ E <0, emission is not isotropic and electrons are only produced within a ‘cone’ of angle along + z , with minimal coupling to transverse momentum components until Δ E ≈0 (ref. 21 ). This is where the coldest electrons are produced. We see a near-constant emittance below threshold, limited by the extraction process, which we measured to be ε r =538±26 nm rad for femtosecond excitation and ε r =141±7 nm rad for microsecond excitation. We attribute the larger emittance for femtosecond excitation to space-charge repulsion because the shorter bunches will have higher charge density. Electron bunches produced with microsecond excitation have a pulse length of 5 ns (bunch length 10 cm), so that space-charge dilution of the emittance will be negligible. For electron pulses of order 150 ps (bunch length 3 mm), and the same total charge, the density increases by a factor of 30 and space-charge effects become significant (see Methods). We see the emittance increasing just below field-free threshold (region i of Fig. 4 ), which coincides with an observed increase in ionization efficiency. With increased energy, β c →0 and electrons can be emitted along − z leading to significant scattering from the ion, resulting in an increase in velocity spread and emittance. The increase in efficiency is due to the overlap of accessible emission angles and the polarization-dependent dipole interaction between the electron and ionization laser. With a greater ionization efficiency, any space-charge effects will be exacerbated. For energies above field-free threshold, the emittance with microsecond excitation is mostly consistent with equation (6). For femtosecond excitation, we observe dramatic growth in the spread of emittance values measured in the region around the field-free threshold (region ii of Fig. 4 ). Each individual emittance measurement (see Methods) has a small uncertainty, and large error bars are indicative of a large range of measured emittance values. The increased spread in emittance values above threshold is attributed to opening of an alternative ionization pathway. In the region below threshold, the ionization laser couples the 5P 3/2 state to one or more field-ionising Rydberg states, resulting in an electron bunch with minimal energy spread. When the energy of the ionization laser is increased such that it is sufficient to directly couple the 5P 3/2 state to the continuum, the large near-resonant bandwidth of the excitation pulse substantially increases the energy spread. With further increase in energy, we observe a decrease in emittance, matching the predicted value. This shows that the bandwidth of the femtosecond laser is not appreciably contributing to the energy spread. The theoretical plot of equation (6) assumes that any emittance growth is exclusively due to the excess energy from the ionization laser, without inclusion of space-charge effects, or the heating processes during ionization and extraction (see Methods). Measurement of emittance when the beamlets are created at the source imposes an upper limit to the emittance of an electron beam with any source size. Except for the case of a uniform ellipsoidal bunch, the greatest emittance growth occurs at the beam edges [22] . The emittance measured with the pepper-pot at the source is therefore greater than the emittance one would measure if the whole atom cloud was ionized, and the emittance measured with a mechanical pepper-pot mask at some point downstream. In addition, for low current beams, creating the beamlets at the source allows the emittance growth of the entire electron transport system to be characterized. Electron source shaping via spatial modulation of the excitation laser beam not only facilitates source diagnostics but can also allow for the creation of uniformly distributed ellipsoidal bunches, with linear internal Coulomb fields. Ellipsoidal bunches preserve their initial linearity in phase space, meaning the Coulomb expansion can be completely reversed with linear optics and without degradation of coherence [22] . With such bunches, the brightness is then limited by the initial phase-space density of the source. Careful characterization and optimization of the initial emittance is vital, and the unique shaping abilities of a CAES allow these measurements and optimization to be performed in real time. Combination of electron bunch shaping and two-colour photoionization allows for creation of the ideally distributed sub-260 ps electron pulses, which are suitable not only for UED but also for injection into particle accelerators, synchrotrons and free-electron lasers [23] . We have shown that two-colour photoionization allows generation of electron bunches that are both short and highly coherent, despite the spectral width of the ultrafast excitation laser pulse. When atoms are field ionized from Rydberg states, anisotropy in the energy distribution results in electron bunches with minimal transverse emittance. An upper limit to the source emittance of ε r =538±26 nm rad was measured, corresponding to a coherence length of L c =4.0±0.2 nm, sufficient for imaging nanocrystals. During preparation of this manuscript, we became aware that similar results have been obtained using slow excitation at 780 nm and femtosecond ionization at 480 nm ( [24] ). The creation of cold, ultrafast electron bunches by either method provides a promising way forward for UED imaging. Experimental apparatus and techniques A rubidium-85 magneto-optical trap of approximately 10 9 atoms trapped in a 5-mm diameter region was loaded from a Zeeman slower [25] attached to an effusive atom source. A quasi-mirror magneto-optical trap design was used, with a conductive mirror to reflect four of the cooling beams and to form one accelerator electrode. The other electrode was formed by a transparent conductive window [26] . Trapped atoms were illuminated by an excitation laser driving the 5S 1/2 ( F =3)→5P 3/2 ( F =4) transition, shaped with a spatial light modulator to form a pepper-pot intensity distribution in the x–y plane. The excited-state atomic distribution in the x–y plane was thus defined by the initial atomic density and the shaped excitation laser intensity. Atoms in the 5P 3/2 state were photoionized by a 5-ns 480-nm laser pulse, focused to a 100 μm × 8 mm (FWHM) ribbon in the x–y plane. At the overlap of the laser beams, atoms were ionized to form a pepper-pot density distribution of electrons and ions, with excess ionization energy primarily determined by the ionization laser wavelength [27] . The initial transverse electron density is determined by the excitation laser profile and atom distribution. Ionization occured in a static acceleration field of 40 kV m −1 . The extracted electrons were incident on a phosphor-coupled microchannel plate, which was imaged with a cooled interline transfer CCD (charge-coupled device) camera. A conservative estimate of the bunch charge is made by assuming saturation by the femtosecond laser such that 50% of illuminated atoms are excited, and ionization of 20% of the excited atoms illuminated by the nanosecond laser, resulting in a 10% net photoionization efficiency. Using the cold atom density and the laser beam waists given above, the electron number is then approximately 6 × 10 5 electrons or 100 fC. Electron beam characteristics Emittance is a measure of the phase-space volume occupied by the electron bunch. The normalized RMS emittance ε x is defined by: where m e is the electron mass, x is the transverse position with x =0 the average position of the bunch and p x is the transverse electron momentum. The brackets ‹…› indicate the ensemble average taken over the electron bunch. Experimentally, we determine the momentum spread from measurement of the angular divergence. Defining x ′= v x / v z , and provided v x << v z , which is true for paraxial beams, x ′ is the angle a particle makes with the beam axis of symmetry. Thus, the emittance can be expressed as: where β = v z / c and is the trace-space volume of the beam that is actually measured. For a CAES, we can assume a thermal distribution such that the spatial coherence is given by [28] : where k B is the Boltzmann constant and T is the apparent electron temperature. To observe interference, the coherence length must be of order twice the unit-cell spacing of the sample. At a beam waist, the transverse spatial coherence length is related to the emittance by [12] : where is the RMS bunch radius, and . Combining equations (4) and (5) yields The transverse brightness for a beam with peak current I propagating in the z direction can be defined as [29] : which is fundamentally limited by the phase-space density of the source. Thus, measurement of the source emittance allows determination of both the spatial coherence length (equation 5) and the source brightness (equation 7). The pulse length was estimated from the physical dimensions of the overlap of the excitation and ionization laser beam profiles at the cold atom cloud, and the potential gradient of the accelerator. Defining the centre of the atom cloud to be at position d along the propagation axis, and the detector to be at p , the time of flight for an electron formed at time t 0 and position δ relative to the cloud centre to reach the detector is t = t 0 +( d −2 δ + p )/ v ( δ ) where the velocity . The 3 σ pulse duration is then 150 ps. Pepper-pot analysis A 3 × 3 pepper-pot pattern was used with sufficient separation to ensure no overlap between beamlets in the detector plane at higher ionization energies, a condition required for analysis. For femtosecond excitation, the aperture separation was x pp =1.9 mm with each ‘aperture’ having a measured FWHM of μm. For microsecond excitation, x pp =1.5 mm and μm. The dependence of excess ionization energy on the emittance was investigated by repeating the same measurements at varying ionization laser wavelengths, shown in Fig. 4 . The theoretical emittance values were calculated from equation 6, where k B T has been replaced by Δ E ( λ ) from equation 1 and the values for σ r are calculated from x pp . The method of spatial light modulator phase mask production for producing arbitrary laser intensity distributions is outlined in McCulloch et al . [11] . The binary transmission function of the pepper-pot was modulated to compensate for the atomic density profile of the cold atom cloud to form uniform-density electron beamlets upon ionization. The increase of the electron beam emittance with propagation due to space-charge-driven expansion is significant if the Debye length λ D =( ε 0 γk B T / e 2 n ) 1/2 << σ r ( [29] ). For the nanosecond bunches, λ D ≈50 σ r and space-charge effects are negligible. For the picosecond bunches within each beamlet at the MCP plane, λ D ≈5 σ r and space-charge interactions therefore make a significant contribution to the measured emittance. How to cite this article : McCulloch, A. J. et al . High-coherence picosecond electron bunches from cold atoms. Nat. Commun . 4:1692 doi: 10.1038/ncomms2699 (2013).